Magnetic force microscopy reveals meta-stable magnetic domain states that prevent reliable absolute palaeointensity experiments Obtaining reliable estimates of the absolute palaeointensity of the Earth’s magnetic field is notoriously difficult. The heating of samples in most methods induces magnetic alteration—a process that is still poorly understood, but prevents obtaining correct field values. Here we show induced changes in magnetic domain state directly by imaging the domain configurations of titanomagnetite particles in samples that systematically fail to produce truthful estimates. Magnetic force microscope images were taken before and after a heating step typically used in absolute palaeointensity experiments. For a critical temperature (250 °C), we observe major changes: distinct, blocky domains before heating change into curvier, wavy domains thereafter. These structures appeared unstable over time: after 1-year of storage in a magnetic-field-free environment, the domain states evolved into a viscous remanent magnetization state. Our observations qualitatively explain reported underestimates from otherwise (technically) successful experiments and therefore have major implications for all palaeointensity methods involving heating. Our understanding of both long- and short-term geomagnetic behaviour depends on the availability of reliable well-dated full-vector descriptions of the Earth’s magnetic field [1] , [2] . Such records—preferably evenly distributed over the globe—consist of both palaeodirections and palaeointensities. Directional information is generally straightforward to obtain from various recorders, including well-dated lavas and (lake) sediments for shorter timescales and sedimentary sequences for reconstructions going further back into geological history. Despite recent methodological progress [3] , [4] , [5] , [6] , [7] , [8] , [9] , [10] , [11] , [12] , however, acquiring reliable absolute palaeointensity data remains a formidable task. Only materials that acquired their remanent magnetization by cooling in the Earth’s ambient magnetic field are suited for absolute palaeointensity determinations. Therefore baked archaeological artefacts and igneous rocks are the only reliable recorders available. Archaeological artefacts, however, are linked to ancient civilizations and their availability is therefore limited to specific ages and locations; to obtain records well-distributed around the globe and extending beyond the realm of ancient civilizations, we have to unlock the archive of extrusive igneous rocks. In samples that are suitable for absolute palaeointensity techniques, the natural remanent magnetization (NRM) imparted by the unknown ambient field at the time of cooling must be a thermo-remanent magnetization (TRM). This primary TRM is then compared with a laboratory-imparted partial TRM (pTRM) in a known magnetic field. Palaeointensity techniques therefore rely on the assumption that the pTRMs are acquired analogously to the NRM of the samples, which is valid only for very small magnetic grains [13] , [14] that are single domain (SD), as typically found in baked archaeological artefacts [15] . Larger grains, however, are divided into more magnetic domains separated by domain walls; the NRM configuration of these magnetic domains is not necessarily reproduced after imparting a pTRM. The remanence in lavas is unfortunately often carried by such ‘pseudo-single domain’ (PSD) or ‘multidomain’ (MD) grains, and MD or ‘transdomain’ processes therefore often prevent reliable palaeointensity experiments on extrusive igneous rocks [16] , [17] . Over the past decades, various tests and protocols have been proposed to identify and (partially) overcome the MD effects during palaeointensity experiments [3] , [4] , [5] , [6] , [7] , [8] , [9] , [10] , [11] , [12] , but success rates of such experiments are still notoriously low [17] , [18] , [19] , [20] . It is even more disturbing that—in spite of extensive testing—palaeointensity experiments sometimes yield technically successful estimates of the palaeofield that actually over- or underestimate the palaeofield by tens of percent [6] , [21] . Historical flows from Mt. Etna (Italy) have been extensively studied in terms of absolute palaeointensity before, with several different methods and techniques [3] , [21] , [22] , [23] , [24] , [25] , [26] , and are renowned for their difficulty to deliver faithful palaeointensities. Different palaeointensity protocols, such as the IZZI [7] , [8] and Aitken [27] Thellier experiments; the microwave Thellier protocol [3] ; and the multispecimen-style [9] , [10] technique generally yield distinct underestimates of the palaeofield of up to ~45% (refs 3 , 21 , 26 ). Even Thellier results passing a strict set of selection criteria, PICRIT-03 (ref. 28 ), yield an average underestimate of 16% (ref. 21 ); for the multispecimen-style palaeointensity techniques underestimates of 30–45% of the palaeofield are reported [26] . To uncover why certain lavas systematically fail to deliver faithful palaeointensities, we directly imaged changes in domain configurations in a typical historical flow from Mt. Etna after imparting a pTRM at three different temperatures using magnetic force microscopy (MFM). At a temperature typically exploited in palaeointensity experiments for these samples (250 °C) the grains reveal major changes in the type of magnetic domain configuration in their pTRM state. These pTRM domain states proved to be meta-stable over time: the domain configuration evolved to a viscous remanent magnetization (VRM) state after 1-year storage in a magnetic-field-free environment. The observed meta-stable domain configurations after heating to 250 °C qualitatively explain underestimates often found in technically successful palaeointensity experiments for the type of lava subjected to this study. Magnetic force microscopy MFM was selected to visualize the magnetic domains because of its resolution and relative ease of use. Up to now this technique has been mainly adopted in fundamental magnetic property studies [29] : it was used to image the classical domain configurations (180°, 109° and 71° walls with closure domains and Néel caps) in MD magnetites [30] , [31] , [32] , [33] . Naturally occurring titanomagnetites, however, have rarely been studied. Here, we image magnetic domains of titanomagnetite grains while still embedded in the constituting lava. Our experimental procedure is rather straightforward: we take MFM images of grains in their pristine NRM state and after imparting a pTRM. The samples were then stored in a magnetic-field-free environment for 1 year, after which the same grains were scanned again using the MFM technique. With this approach it is possible to visualize potential changes in domain configuration over time. One sample was imaged after imparting a pTRM at 120 °C, a second at 250 °C and a third at 450 °C. At 120 °C, domain walls should not be unblocked significantly as was indicated by our rock-magnetic experiments; only ~10% of the NRM is unblocked at this temperature. This 120-°C step is primarily chosen as a check for the routine of preparing the samples, imparting the pTRM and obtaining MFM images: if domain walls are shifted or changed on a large scale after heating to this temperature the magnetization of the grains is affected by sample handling or processing during the various steps of the experiment. We selected 250 °C as a temperature typically exploited in palaeointensity experiments for these samples: Thellier [7] , [8] palaeointensity experiments were interpreted between 100 and 280 °C (ref. 26 ) while multi specimen style (MSP) experiments [9] , [10] were done at 250 °C (ref. 26 ). The highest temperature used here is 450 °C, well above the temperature at which severe alteration occurs as indicated by our rock-magnetic analyses. We included this temperature to assess the influence of thermochemical alteration on the domain states in our samples. Sample material We selected a site from the Mt. Etna 1971 flow for this study (site ET-71-2A [26] ), because it failed to produce reliable palaeointensities in spite of careful testing by several groups [3] , [21] , [22] , [26] . Furthermore, this site thermochemically represents ~50% of all Mt. Etna lavas (see Methods). Optical and scanning electron microscopy ( Figs 1 and 2 , respectively) reveal two distinct generations of titanomagnetite grains in our samples [21] , [22] . One generation consists of large grains, tens to hundreds of micrometres in size, with well-developed oxyexsolution lamellae, corresponding to oxidation class C4 to C6 of Haggerty [34] . They either are xenocrysts, or they were formed during very slow cooling in the magma chamber [21] . The volumetric majority of the grains, however, is distinctly smaller (<20 μm), and shows little signs of oxidation corresponding to Haggerty’s oxidation class C1 to C2 ( Fig. 2 ; Supplementary Fig. 1 ). These grains are therefore from a later generation of titanomagnetites that formed during emplacement of the lava. 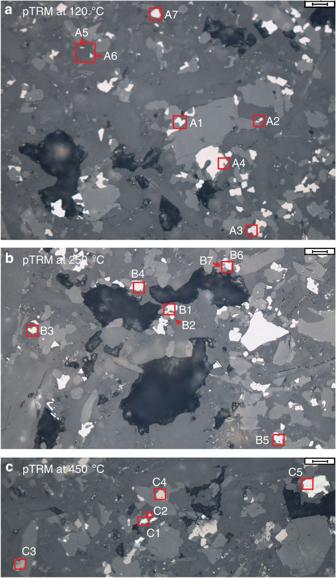Figure 1: Optical microscope images of the samples used in this study. The three samples were subjected to pTRMs at different temperatures: 120 °C (a); 250 °C (b); and 450 °C (c). The grains that were analysed with the MFM are indicated by the red squares (and/or arrows). The two biggest grains, A4 and C5 show oxyexsolution lamellae and correspond to the first generation of titanomagnetites21,22. Grains A1, B5 and B6 are also oxidized, as revealed by microprobe analyses. All oxidized grains show signs of resorption on the edges of the grains. Smaller grains, that is the second-generation titanomagnetites, have unoxidized compositions. The scale bars in the upper right corners of the panels are 20 μm. Figure 1: Optical microscope images of the samples used in this study. The three samples were subjected to pTRMs at different temperatures: 120 °C ( a ); 250 °C ( b ); and 450 °C ( c ). The grains that were analysed with the MFM are indicated by the red squares (and/or arrows). The two biggest grains, A4 and C5 show oxyexsolution lamellae and correspond to the first generation of titanomagnetites [21] , [22] . Grains A1, B5 and B6 are also oxidized, as revealed by microprobe analyses. All oxidized grains show signs of resorption on the edges of the grains. Smaller grains, that is the second-generation titanomagnetites, have unoxidized compositions. The scale bars in the upper right corners of the panels are 20 μm. 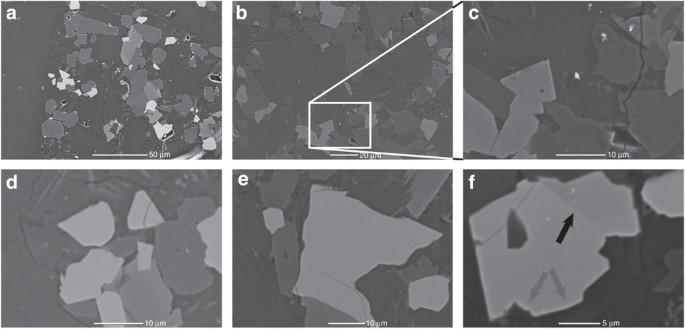Figure 2: Scanning electron microscope images of site 71–2A. Panelsa–care taken in secondary electron mode for better contrast between the grains and grain size analyses; panelsd–fare taken in backscatter electron mode to emphasize features within the grains such as signs of oxidation. The iron oxides are easily identified as brighter particles. The smallest iron oxide grains present (c) are in the order of 1 μm in diameter, well above the resolution limit of the scanning electron microscope None of the second-generation iron oxides (d,e) show signs of either high- or low-temperature chemical alteration63(that is, cracked or blurred edges, zoning, lamellae and so on) at any of the magnifications used. One of the large particles (f), however, reveals some zoning (black arrow), and a bright edge (grey arrows)—signs of moderate oxidation. Because of its size and signs of oxidation, this grain is classified as being from the first generation of titanomagnetites present in the sample. The length of the scale bars for panelsa–fis, respectively, 50, 20, 10, 10, 10 and 5 μm. Full size image Figure 2: Scanning electron microscope images of site 71–2A. Panels a – c are taken in secondary electron mode for better contrast between the grains and grain size analyses; panels d – f are taken in backscatter electron mode to emphasize features within the grains such as signs of oxidation. The iron oxides are easily identified as brighter particles. The smallest iron oxide grains present ( c ) are in the order of 1 μm in diameter, well above the resolution limit of the scanning electron microscope None of the second-generation iron oxides ( d , e ) show signs of either high- or low-temperature chemical alteration [63] (that is, cracked or blurred edges, zoning, lamellae and so on) at any of the magnifications used. One of the large particles ( f ), however, reveals some zoning (black arrow), and a bright edge (grey arrows)—signs of moderate oxidation. Because of its size and signs of oxidation, this grain is classified as being from the first generation of titanomagnetites present in the sample. The length of the scale bars for panels a – f is, respectively, 50, 20, 10, 10, 10 and 5 μm. Full size image Since the remanent magnetization in our samples is carried by titanomagnetites of various grain sizes and from two generations, it is important to assess which grains constitute the majority of the bulk magnetic remanence. From the scanning electron microscopy images, we can derive the grain size distribution in our samples, although we acknowledge that very small grains ( ≪ 0.5 μm) may be underestimated in the image analyses ( Supplementary Figs 2 and 3 ). The grain size distributions peak at ~1–1.5 μm ( Supplementary Figs 2 and 3 ) and show a distinct decline for smaller sizes that are, however, well within the range where meaningful size analysis is possible. For magnetite (TM-0) the relation between grain size and contribution to the bulk TRM intensity is relatively well constrained [35] . If this relation can also be applied to titanomagnetite, the contribution of small, SD grains (<2 μm) to the bulk magnetization of our samples is <~10% ( Supplementary Figs 2 and 3 ). The majority (~70–80%) of the magnetic remanence is carried by PSD to MD grains of the second generation of titanomagnetites (2–20 μm). Furthermore, small, SD grains are both theoretically [13] , [14] and empirically [15] known to yield good results in palaeointensity experiments; erroneous palaeointensity results are often attributed to transdomain processes in larger grains. We therefore choose to image 5–7 grains per sample ranging between 2 and >20 μm—in the PSD to MD range. These second-generation titanomagnetite grains are discussed in the main text; images of grains that show distinct oxyexsolution lamellae and grains for which oxidation is indicated by the chemical analyses ( Supplementary Table 1 )—that is, grains from the first generation of titanomagnetites—are in Supplementary Figs 4, 5 and 6 . Rock-magnetism and palaeointensities The rock-magnetic experiments ( Supplementary Fig. 7 ) indicate that samples from the selected site should be very suitable for palaeointensity experiments. They contain a suite of PSD titanomagnetites with a broad range of Curie temperatures, and their magnetic properties are not irreversibly altered thermochemically before reaching 320 °C. Yet, >50% of the NRM is unblocked at 250 °C ( Supplementary Fig. 7 ). The palaeointensity results for the site selected for this study underestimate the expected palaeofield by 11.6% (Aitken-Thellier [27] ) and 43.3% (domain state corrected multi specimen method (MSP-DSC) [9] , [10] ) [26] ( Supplementary Fig. 8 ). However, both the Thellier and MSP-DSC results obtained from this site would normally be rejected, because of their technical quality (Thellier) or failure in the anhysteretic remanent magnetization (ARM)-test [12] (MSP-DSC). Samples heated to 120 °C The domain state of the grains that were heated to 120 °C only shows very minor changes, if changes are present at all ( Fig. 3 ). Domain walls are typically sharp and domains are rectangular in shape. Because the polished surface is not aligned with a crystal lattice plane, domains regularly appear intersected under various angles. Whenever the magnetization has a dominant polar component (vertical to the surface) the MFM image resembles a polar Kerr image [29] and can be compared with images from Ambatiello and Soffel [36] . The best example is the NRM in grain B2 ( Fig. 4 ) that shows clear dark and lighter stripe domains apparently due to a strong polar magnetization. However, it is rarely possible to identify ideal domain structures typical for titanomagnetites in a (110) plane where the magnetization lies within the observation plane [30] , [32] , [36] , [37] , [38] , [39] , [40] . One example may be the NRM state in grain A2, especially its upper right part, where the domains appear uniformly dark, but the domain walls are represented by sharp bright lines corresponding to a domain configuration mainly parallel to the plane of view and polar magnetization in the walls. In most other grains, mixtures of these extreme cases occur, whereby also an overlay of distinct closure domain patterns above a more diffuse volume charge from underlying larger domains can occur (c.f. Hubert and Schäfer [29] , p. 437). The domain patterns observed in grains A5 and A6 show some differences already after heating to 120 °C ( Fig. 3 ). However, in both cases the underlying large-scale pattern appears unchanged, while newly nucleated domains with a strong polar magnetization emerge. These two grains are relatively rich in Ti, and their Curie temperature may therefore be lower and domains more easily unblocked. Easy nucleation of new closure domains out of the NRM state could also be a side effect of a volume change during polishing. 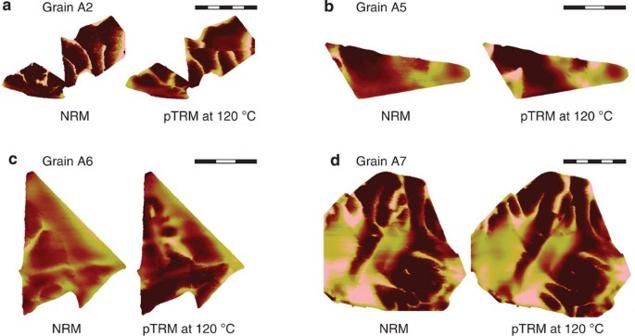Figure 3: Grains in the sample subjected to a pTRM at 120 °C. (a–d) Four typical grains in their NRM state (left-hand side images) and pTRM state (right-hand side images). Domain structures hardly change; especially in grains A2 (a) and A7 (d) the configuration is remarkably similar in the pTRM state. Grains A5 (b) (in its lower left corner) and A6 (c) (in the centre) do show minor changes, however. The chemical analyses (Supplementary Table 1) indicate a relatively high Ti-content for these grains, lowering their Curie temperature. Scale bar, 5 μm (a,d); 3 μm (b,c). Figure 3: Grains in the sample subjected to a pTRM at 120 °C. ( a – d ) Four typical grains in their NRM state (left-hand side images) and pTRM state (right-hand side images). Domain structures hardly change; especially in grains A2 ( a ) and A7 ( d ) the configuration is remarkably similar in the pTRM state. Grains A5 ( b ) (in its lower left corner) and A6 ( c ) (in the centre) do show minor changes, however. The chemical analyses ( Supplementary Table 1 ) indicate a relatively high Ti-content for these grains, lowering their Curie temperature. Scale bar, 5 μm ( a , d ); 3 μm ( b , c ). 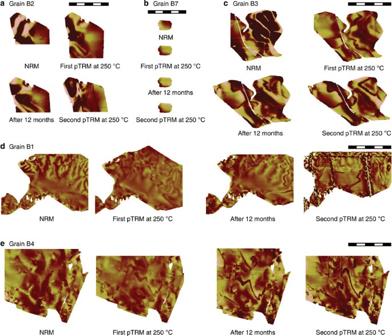Figure 4: Grains in the sample subjected to a pTRM at 250 °C. All scale bars are 5 μm. Four images are given per grain analysed: (1) the MFM image of the grain in its NRM state; (2) an image of the grain in its pTRM state; (3) the domain configuration after storing the samples for 1 year in a magnetic-field-free environment after the first pTRM was acquired; and (4) an image of the domain configuration after imparting a second pTRM. Except for the smallest grain analysed (B7) (b), all grains change the type of domain configuration from blocky, rectangular domains in the NRM state to curvy domains that in some grains appear as shells in their pTRM state (a,c,d,e). Furthermore, domain walls are less distinct, therefore probably wider, in the pTRM state compared with the NRM state. This is best illustrated by the right half of grain B3 (c). This new domain configuration, however, is not stable over time: after 1 year, domains become more rectangular in shape and domain walls more distinct, as visualized in the centre of grain B1 (d) and grain B4 (e). The second pTRM partly restores the curvy domains, although sample B1 was scratched (black dashed lines) in the process of imparting the second pTRM, and closure domains are evident at the scratches. The smallest grain in this study, B7 (b), shows only two domains that flip polarity in the first pTRM state; this state is stable over time and repeated by the second pTRM imparted. Full size image Figure 4: Grains in the sample subjected to a pTRM at 250 °C. All scale bars are 5 μm. Four images are given per grain analysed: (1) the MFM image of the grain in its NRM state; (2) an image of the grain in its pTRM state; (3) the domain configuration after storing the samples for 1 year in a magnetic-field-free environment after the first pTRM was acquired; and (4) an image of the domain configuration after imparting a second pTRM. Except for the smallest grain analysed (B7) ( b ), all grains change the type of domain configuration from blocky, rectangular domains in the NRM state to curvy domains that in some grains appear as shells in their pTRM state ( a , c , d , e ). Furthermore, domain walls are less distinct, therefore probably wider, in the pTRM state compared with the NRM state. This is best illustrated by the right half of grain B3 ( c ). This new domain configuration, however, is not stable over time: after 1 year, domains become more rectangular in shape and domain walls more distinct, as visualized in the centre of grain B1 ( d ) and grain B4 ( e ). The second pTRM partly restores the curvy domains, although sample B1 was scratched (black dashed lines) in the process of imparting the second pTRM, and closure domains are evident at the scratches. The smallest grain in this study, B7 ( b ), shows only two domains that flip polarity in the first pTRM state; this state is stable over time and repeated by the second pTRM imparted. Full size image Samples heated to 250 °C All grains in the sample heated to 250 °C show notable changes in the structure of the domains in their pTRM state ( Fig. 4 ). Generally, sharp domain walls and rectangular-shaped domains characteristic of the NRM state change into more diffuse wavy domain patterns with less distinct walls. These changes are most evident in the larger grains (>8 μm). The clearest example is grain B3: the distinct, blocky domains of the NRM state change into a configuration that appears to reflect wavy, circular domains akin to Fig. 5d in Ambatiello and Soffel [36] . In B3, these wavy domains are typically <1 μm wide and a few μm long. The smallest grain included in this study, B7, is ~3 μm in diameter and shows only two domains, which is consistent with Fig. 7 of Ambatiello and Soffel [36] . After imparting the pTRM, the domains of grain B7 flip polarity, while retaining their overall shape, which indicates that the domain structure is strongly confined by either particle shape [41] or internal stress. 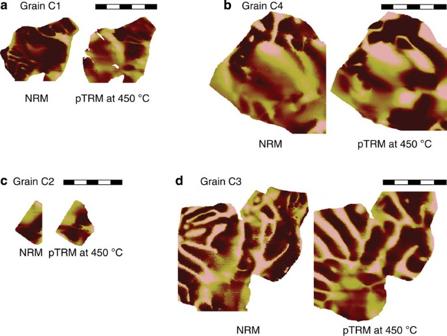Figure 5: Grains in the sample subjected to a pTRM at 450 °C. Again, the images of the grains in their NRM state on the left and the images of the grains in their pTRM state on the right. All scale bars are 5 μm. Changes are evident, as expected after heating the grains well above their alteration temperature, as indicated by the susceptibility-versus-temperature experiments (Supplementary Fig. 7). Domains tend to become larger in the pTRM state, and domain walls more distinct (b,d). This behaviour is most evident in the upper left-hand corner of grain C3 (d), where narrow NRM domains change their orientation by ~90°. The smaller grains, C1 and C2 (aandc, respectively), appear less affected by the alteration at high temperatures, better reproducing the NRM domain state than the larger grains. However, the curvy domain configurations as observed in the grains heated to 250 °C (Fig. 3), are not seen here. Figure 5: Grains in the sample subjected to a pTRM at 450 °C. Again, the images of the grains in their NRM state on the left and the images of the grains in their pTRM state on the right. All scale bars are 5 μm. Changes are evident, as expected after heating the grains well above their alteration temperature, as indicated by the susceptibility-versus-temperature experiments ( Supplementary Fig. 7 ). Domains tend to become larger in the pTRM state, and domain walls more distinct ( b , d ). This behaviour is most evident in the upper left-hand corner of grain C3 ( d ), where narrow NRM domains change their orientation by ~90°. The smaller grains, C1 and C2 ( a and c , respectively), appear less affected by the alteration at high temperatures, better reproducing the NRM domain state than the larger grains. However, the curvy domain configurations as observed in the grains heated to 250 °C ( Fig. 3 ), are not seen here. Full size image The observed pTRM domains are not stable over time. After storing the sample for 1 year in a magnetic-field-free environment the domain walls typically became more distinct and less wavy in shape, and thus more closely resembled the initial NRM appearance. This is well illustrated by grains B1 and B3: the domains in the middle of grain B1 have become larger and more rectangular in shape; in B3, the domain walls are more distinct. After imparting a second pTRM at 250 °C the domains again seem to be wavier and domain walls less distinct. However, the changes after the second pTRM appear less marked with respect to the NRM state than the changes after imparting the first pTRM. A common observation is that the first pTRM substantially rearranges the NRM domain state, while retaining typical stress or shape-induced patterns of the domain configuration. The resulting configuration shows less contrast in MFM images, probably owing to a major contribution from more distant volume charges that reflect larger domain configurations. After 12 months a more diversified domain structure with domains closer to the surface has formed, which appears sharper and produces a stronger contrast in the MFM images. The second pTRM then leads to a less marked domain rearrangement, but also removes the more distinct near-surface structures. Samples heated to 450 °C In the samples heated to 450 °C, well above the alteration temperature as determined by preceding rock-magnetic analyses ( Supplementary Fig. 7 ), the domain configurations of the titanomagnetite grains can change markedly ( Fig. 5 ). Besides the magnetization orientation, also stress or shape-induced features in the NRM state can change substantially. For example, the orientation of the domains on the left-hand side of grain C3 is rotated by ~90°. Only the small grain (C2, <5 μm) largely retains its NRM domain configuration. Interestingly, the more curvy, diffuse appearance of domains, as observed in the pTRM state of the grains heated to 250 °C, is not observed in the grains heated to 450 °C. This may hint to an increase of internal stress, whereby more distinct, stress-dominated domain structures with fewer surface closure domains are formed. The observed processes after heating the sample to 450 °C may be akin to the irreversible thermomagnetic behaviour as observed by Bowles et al. [42] , and attributed to cation reordering in titanomagnetites induced by heating. Hard magnetic MFM tips can alter the magnetic state of soft magnetic samples [43] , [44] . To test the veracity of MFM imaging on our samples, we acquired MFM images of grains after removing and re-inserting the sample, and after rotating the sample by 90°. None of these actions changed the domain configuration observed in the grains. The magnetic state of our samples is therefore not noticeably altered by the MFM procedure itself, and sample–tip interaction induces negligible changes. Besides confirming the validity of our domain observations, this also indicates that the titanomagnetite domain configurations are not easily moved. Our observations concur with the classification of TM-50 to TM-60 (Fe 2.5 Ti 0.5 O 4 —Fe 2.4 Ti 0.6 O 4 ) as being magnetically hard owing to large magnetostrictive anisotropy and relatively low saturation magnetization ( M S ) [45] . As expected, the grains in the sample that were heated to 120 °C did not show large-scale changes in domain configuration. Therefore, we conclude that all steps in the experimental procedure—obtaining MFM images, encapsulating the samples in an evacuated glass tube, imparting the pTRM and taking MFM images again—do not interfere with the magnetic state of the sample. Furthermore, the silica colloid suspension polish (see Methods) properly removes potential surface stress induced by the mechanical polishing, since the thermal step at 120 °C would at least partially remove the surface stress (see Supplementary Fig. 9 for a MFM image of a stressed surface). After heating to 250 °C the blocky, rectangular domain shapes with distinct domain walls are replaced by wavy domains with smoother edges. Wavy domain patterns were observed previously in large MD titanomagnetites (TM-60) using Bitter patterns at room temperature [37] . Those patterns were explained by high degrees of stress (50–100 MPa; 0.5–1.0 kbar) in those particular samples, but were later attributed to a large magnetic component normal to the plane of view [38] . Furthermore, wavy domains in titanomagnetite have been linked to spike or wedge-shaped closure domains [36] . MFM images of grains in which the surface stress induced by the mechanical polishing was not sufficiently removed sometimes also show such small-scale wavy patterns at room temperature ( Supplementary Fig. 9 ). Néel [14] introduced the concept of local energy minimum (LEM) states in 1955 (refs 46 , 47 , 48 ); it is predicted that grains do not always occupy their absolute energy minimum. The domain configuration of a particle is the expression of its magnetic energy state, and a specific grain has the choice between several LEM states depending on its thermomagnetic history. Halgedahl [38] found LEMs to be remarkably stable when the grains were heated to their respective Curie temperatures, and suggested that the energies that drive domain transitions give random access to a range of LEM states separated by comparatively low energy barriers at temperatures near the Curie point. Small differences in the thermomagnetic history can then influence the thermal evolution of the domain structure. The Curie temperatures of the grains analysed after heating to 250 °C are derived from their chemical composition [49] ( Supplementary Table 1 ) and are inferred to be slightly lower than 250 °C. To explain the observed differences between the NRM and the pTRM state after heating to 250 °C, we envisage two possible scenarios. In the first scenario, the Curie temperature of the grains is not homogeneously distributed within the grain. Since the temperature used in the experiments is within 10 °C of the inferred Curie temperatures for the PSD/MD grains in Fig. 4 , minor compositional heterogeneities may locally lead to slightly higher Curie temperatures. Therefore some domain walls or nuclei may not fully unblock at this temperature. Imperfections in the crystal lattice can pin domain walls [46] , [50] , [51] and thereby force grains to remain in a higher LEM once brought in such a state. The domain walls or domain nuclei that are not unblocked may act similar to imperfections in the crystal lattice and force the grain into a different LEM than the LEM obtained after cooling from above the Curie temperature to room temperature—the process of acquiring the initial TRM, that is, the samples’ NRM. In this scenario, the pTRM state differs from the NRM state because the NRM was not fully removed from the grain. In the second scenario, the grains would be heated to above their Curie temperature and therefore acquire a full TRM during the heating–cooling cycle. This implies that the domain configuration of the full TRM acquired in the laboratory differs from the initial full TRM (that is, the NRM) of the grains, since the conditions in the grain before blocking the magnetic signal during cooling would be equal for the NRM and (p)TRM state (that is, a fully unblocked grain) in this scenario. If applicable, this would have ramifications for the interpretation of the NRM as a pure TRM because time-dependent processes at room temperature would provoke changes. Both Thellier- and multispecimen-style palaeointensity experiments underestimate the palaeofield for the samples subjected to this study. Such underestimates occur if the (p)TRMs induced by the same DC field as the NRM-imparting field are higher than the NRM erased. In this case, the grains possess a larger net magnetic moment in their (p)TRM state. Combining this with the domain observations implies that the curvy, diffuse domain configurations of the (p)TRM states after heating to 250 °C carry higher magnetic moments, and therefore reside in a higher LEM than their previous NRM. A physical mechanism for magnetic domains to change size, position or even entire configurations is provided by the temperature dependence of the magnetocrystalline contribution and magnetostriction contributions. While heating, the magnetocrystalline anisotropy constant ( K 1 ) of Ti-poor titanomagnetite changes [52] . At room temperature, magnetite and TM-60 have the same |K 1 |/M s ratio [53] and the anisotropy in TM-60 is dominated by magnetostriction and intrinsic stress [45] . If the magnetocrystalline contribution is relevant for temperature dependence also in TM-60, the temperature-dependent trends [52] observed in magnetite may be extrapolated to titanomagnetite: the magnetostriction constant for TM-0 linearly decreases between room temperature and the Curie temperature [54] . Such temperature-dependent reconfigurations of magnetic domains occurring during heating and cooling samples in palaeointensity experiments may put the grains in a different LEM than the LEM that stored the NRM, and therefore lead to incorrect palaeointensity estimates. Time-dependent domain reconfigurations—often referred to as viscous or thermally activated processes [35] —have been observed previously by Muxworthy and Williams [39] . They imaged domain walls in large MD titanomagnetites using Bitter patterns at elevated temperature (<100 °C) and in an applied magnetic field of 2±0.1 mT. The domain walls in their samples moved between ‘quasi-static LEMs’; this behaviour was repeatable per grain, but specific domain structures within the grains did not re-occur. In our observations, the first pTRM at 250 °C is higher than the erased part of the NRM since underestimates are obtained from the palaeointensity experiments. Therefore, the grains in the sample must on average reside in a comparatively high LEM state. Over a time span of 12 months, the domain configuration is rearranged and a lower LEM state has apparently been reached. The net magnetic moment of the grains should therefore be lower and closer to the initial NRM after these 12 months. The viscous processes we observe operate on a much longer timescale: Muxworthy and Williams [39] observe quasi-static LEMs changing over hours to days. The elevated temperature in their experiments may have resulted in comparatively rapid viscous processes compared with our observations that pertain to viscous effects occurring at room temperature. Therefore their observations may be analogous to the process we observe. It is important to note, however, that Muxworthy and Williams [39] applied a magnetic field of 2±0.1 mT during their experiments while our samples were kept in a magnetic-field-free environment; the driving energy for the two observed processes may therefore very well differ. The mysterious ‘drawer storage effect’ described by Shaar et al. [55] does operate at the same timescale (and at the same temperature) as the viscous decay in our samples and may very well be an expression of the process we describe. The viscous decay we observe is systematically present, because the samples were kept in a magnetic-field-free environment at room temperature (variation max 5 °C)—well below their Curie temperatures—for 12 months. This process is always related to the formation of more distinct smaller-scale domain features, probably related to near-surface closure domains. Another, remarkable, observation is that after the second pTRM acquisition at 250 °C the domain structure of the VRM state has not been completely reset, but still influences the second pTRM state, which typically more closely resembles the previous VRM than the first pTRM state. This implies that the VRM, although acquired at room temperature, has not been removed by heating to 250 °C and hardly follows a classical Arrhenius-type law for symmetric energy barriers. Instead, it seems plausible that the viscous relaxation process that occurs at room temperature is highly asymmetric: the energy barriers for relaxation into the new states are relatively small, while the barriers necessary to overcome to return to the initial pTRM state are too high, even at the pTRM temperature of 250 °C. Thus, below this maximum temperature the process NRM→pTRM 1 →VRM→pTRM 2 cannot return to the initial pTRM 1 state, which makes the VRM process a kind of trapdoor for the domain configuration. Micromagnetic modelling provides insight in the most feasible LEM for given grains under certain conditions. In small magnetite grains (<1 μm) curved vortex or flower states can occur as the preferred LEM [56] , [57] , [58] , [59] . Even repeated cycles of heating and cooling to the same temperature systematically change the statistical domain state [60] . In the same way, a cycle of heating combined with viscous remanence acquisition due to storage at a room temperature may systematically change the domain state and the statistical remanent magnetization; this further supports the trapdoor concept in viscous LEM reconfiguration in our samples. To qualitatively explain our MFM observations at room temperature after pTRM acquisition from 250 °C, we envisage an energy landscape containing many LEM states of possibly very different energy levels. Higher-energy LEM states can be separated by low barriers from lower-energy LEM’s in line with the reasoning by Halgedahl et al. [37] , [38] . However, the energy barriers are not necessarily symmetric, and viscous processes thus may have a preferred direction. Whether a single particle occupies one of these states is to some degree fortuitous, because lattice defects and/or existing partially unblocked domain walls favour one or the other LEM state. The remanence related to different acquisition processes, however, is a statistical average and behaves much more regularly. On cooling, the energy barriers between the LEM states typically increase. The LEM states at 250 °C control the choice of the LEM state retained at room temperature, because the energy barriers are sufficiently high to impede reconfiguration to another LEM state with a lower energy level during the cooling itself. However, at room temperature thermal activation continues to operate, and over a sufficiently long waiting time the initial pTRM LEM state may evolve into another LEM state if thermal activation can overcome the lowest energy barrier out of the initial LEM state. The observed meta-stable pTRM domains in a higher LEM and the viscous LEM reconfiguration have major implications for all thermal palaeointensity methods. As mentioned before, underestimates are to be expected from domain configurations in a higher LEM with respect to the NRM, and they are observed for both Thellier-style [3] , [21] , [22] , [26] and MSP-style experiments [26] for these lavas. It is disturbing that these meta-stable pTRM states are stable on laboratory timescales, as the features observed in the MFM images do not change over hours or days. The second pTRM in our samples, imparted over the VRM after 12 months, shows a combination of features related to the VRM state and features similar in size and shape as observed in the first pTRM state. The influence of the VRM on the second pTRM states is small—if present at all—when the second pTRM is imparted immediately after the first pTRM, as is usually done during palaeointensity experiments. If this leads to more similar pTRM states, and therefore more stable behaviour during palaeointensity experiments, the technically successful palaeointensity results (including checks) that significantly underestimate the palaeofield—often reported for Mt. Etna—are explained. Since the rock-magnetic conditions leading to the meta-stable pTRM states are not yet fully understood, it is hard to predict which percentage of lavas suffer from this phenomenon. Evidently, underestimates of the palaeofield are reported on a large scale for Mt. Etna. For Hawaii, however, palaeointensity experiments that fail to deliver a proper estimate of the palaeofield are usually overestimates [6] , [61] . Currently it is unknown whether the viscous LEM reconfiguration observed here not only occurs after the acquisition of pTRMs; it may also have its bearing on the acquisition of the NRM (the full TRM) of the samples. If the grains in the sample heated to 250 °C acquire a full TRM during the experiment—that is, the second scenario discussed above, the differences between the NRM (initial TRM) and the first laboratory pTRM may express the differences in domain state directly after cooling (the (p)TRM state) and after the viscous LEM reconfiguration (the NRM state). It should be emphasized that if the NRM would be stabilized over time by a probabilistic process, the magnitude of the stabilized NRM does not necessarily relate directly to the magnitude of the Earth’s magnetic field at the time of cooling, and crucial information to obtain a reliable palaeointensity from those cooling units may be lost. Since the meta-stable pTRM effect hampers obtaining a reliable palaeointensity estimate using thermal methods, it is important to detect its occurrence. None of our rock-magnetic experiments done on the samples used for this study indicated alteration of magnetic properties at 250 °C ( Supplementary Fig. 7 ). Although the technical quality of the Thellier and MSP-DSC results for this particular flow would not be sufficient to accept their results, this flow is typical for the majority of (historical) Mt. Etna flows. Some other Mt. Etna flows, however, do yield technically successful palaeointensity estimates that underestimate the palaeofield. The recently proposed ARM-test [12] , in which ARM acquisitions of sister specimens before and after heating are compared, was able to discriminate between samples yielding underestimates and samples yielding reliable palaeointensity estimates. These differences in ARM behaviour are, however, very subtle and readily removed by an AF demagnetization of the samples before the ARM acquisition. It is possible to visualize changes occurring in the configuration of magnetic domains after thermal treatments using the MFM-imaging technique. For pTRM temperatures typical to palaeointensity experiments (250 °C), we observe a different type of domain configuration in the pTRM state compared with the NRM state: the blocky, rectangular domain states with distinct domain walls of the NRM state change into wavy domains with less distinct domain walls in the pTRM state. Moreover, this pTRM state proved to be meta-stable over a period of 1 year evolving to a VRM state—a process explained as viscous LEM reconfiguration. These meta-stable domain configurations, corresponding to a LEM state higher than the NRM state, explain underestimates often found in technically successful palaeointensity experiments for the type of lava subjected to this study. Whether this viscous LEM reconfiguration not only occurs after the acquisition of a (p)TRM, but also affects the NRM of the sample is currently still enigmatic. Sample material Lavas from Mt. Etna are often divided in three or four groups based on their thermomagnetic behaviour [3] , [21] , [22] , [26] . The groups are referred to as types L, H and C; sometimes a fourth type M is specified. ‘Type L’ samples are characterized by a distinct decrease of the low-field magnetic susceptibility below 150–200 °C. ‘Type H’ samples retain high susceptibilities above 400 °C. Samples with one distinct Curie temperature in between the types L an H are sometimes labelled as ‘type M’. Combinations of types L, M and/or H are referred to as ‘type C’. Typically ~50% of all recent Mt. Etna lavas sampled belong to this latter group. For the present study, we selected samples of thermomagnetic type C from site ET-71-2 A [26] , sampled from a flow emplaced by the 1971 eruption at the Eastern flank of Mt. Etna (latitude: 37° 44′ 53.63′′, longitude: 15° 5′ 57.36′′). The solid part of this flow is ~1.5 m thick; palaeomagnetic drill cores were taken 33 cm from the top of the solid part. Sample preparation Three polished surfaces were prepared from one typical palaeomagnetic drill core. The top surfaces of these disks (~5 mm radius, 1 mm thick) were polished with a colloid silica suspension (‘Syton polish’) for 1 h to reduce the surface stress induced by the mechanical polishing. Because the grains are randomly oriented in the lava, the polished surfaces are not aligned with a specific crystal lattice plane as is rather common in fundamental magnetic property MFM studies of (titano)magnetite crystals [30] , [32] , [39] . Accordingly, magnetic closure domains will be prominent in the surface magnetization structures. In our study, we imaged five to seven grains in each sample using the MFM technique ( Fig. 1 ; Supplementary Table 1 ). The distance between the grains analysed is typically tens to hundreds of μm to exclude direct magnetic interaction between the grains. The chemical composition of all grains was analysed using a JEOL Microprobe ( Supplementary Table 1 ). From these measurements it may be inferred whether or not the particles are partially oxidized (maghemitized). The majority of the grains analysed range between 3 and 15 μm in size and show minimal signs of oxidation. The titanomagnetite composition of the unoxidized grains is typically TM-52±5 (Fe 2.48 Ti 0.52 O 4 ), implying that the Curie temperature of these grains varies between ~200 and ~300 °C [35] ; this concurs with the Curie temperatures observed in the rock-magnetic analysis ( Supplementary Table 1 ). Apart from the Ti-substitution, between 5 and 10% of the Fe in the titanomagnetite is substituted by mostly Al and Mg, further lowering the Curie temperatures of the grains [62] . The Curie temperatures listed in Supplementary Table 1 pertain to unoxidized titanomagnetite with only Ti-substitution. These are therefore considered upper bounds; the actual Curie temperatures may be slightly lower. Some large grains, that is, A4 and C5, show some well-developed oxyexsolution lamellae (~1 μm wide and up to 10 μm long); some other grains (A1, B5 and B6) are inferred to be also oxidized, but lamellae are not present. All these large grains can be correlated to the first titanomagnetite generation [21] , [22] ( Supplementary Figs 4, 5 and 6 ). MFM A commercially available atomic/magnetic force microscope was used to take the MFM images (Veeco Nanoscope IIIa), with MFMR probes (MFM—reflex coating, hard magnetic tip, tip radius<50 nm; force constant 2.8 N m −1 ; resonance frequency ~75 kHz). The MFM was used in interleave mode: each trace and retrace were analysed first in tapping mode to image the topography of the sample, and second in lift mode (lift height 40 nm) to assess the stray magnetic field perpendicular to the polished surface. The MFM images are obtained in phase-mode. The driving frequency was tuned automatically; the driving amplitude was kept as low as possible to avoid resonance. The resulting images, consisting of 512 traces of 512 pixels (pxs), accordingly reflect smoothed distributions of magnetic surface and volume charges (Hubert and Schäfer [29] , p. 80). The largest area that can be imaged is 14.8 × 14.8 μm. This implies a lowest possible resolution of ~30 nm per px, some small grains are imaged at higher resolution up to ~16 nm per px. Therefore, the resolution limit in all cases is due to the smoothing effects of tip radius and lift height. The colour scale in the images was set by the software (between 5 and 10°) and adjusted manually if anomalous points hampered a proper automatic setting. After obtaining MFM images of the NRM state, the samples were encapsulated in an evacuated glass tube to impart the pTRMs. The NRM direction of the samples was aligned with the furnace field direction in an ASC TD-48SC thermal demagnetizer. The DC field strength was 44 μT, the historic palaeofield in which the samples acquired their NRM. This procedure of imparting a pTRM in the samples is often used in absolute palaeointensity protocols, such as Thellier- and multispecimen-style protocols. Within hours after imparting the pTRMs the very same grains for which MFM images of the NRM state were taken, were imaged again. The type of configuration of the domains in the grains that acquired their pTRM at 250 °C is different than those heated to 120 and 450 °C: blocky, rectangular domains change into wavier domains. To test the stability of these domain structures, we stored the sample heated to 250 °C in a magnetic-field-free environment (ambient field<~100 nT) and took MFM images of the same grains again after 1 year. Finally, to assess the influence of a second pTRM as typically applied in Thellier- and multispecimen-style experiments, the sample that was heated to 250 °C and stored for 1 year was again encapsulated in an evacuated glass tube and subjected to a second heating step to 250 °C, with the furnace DC field of 44 μT in the direction of the NRM/first pTRM. Again, the same grains were imaged using MFM. How to cite this article: de Groot, L. V. et al. Magnetic force microscopy reveals meta-stable magnetic domain states that prevent reliable absolute palaeointensity experiments. Nat. Commun. 5:4548 doi: 10.1038/ncomms5548 (2014).